Direct observation of the oxygenated species during oxygen reduction on a platinum fuel cell cathode The performance of polymer electrolyte membrane fuel cells is limited by the reduction at the cathode of various oxygenated intermediates in the four-electron pathway of the oxygen reduction reaction. Here we use ambient pressure X-ray photoelectron spectroscopy, and directly probe the correlation between the adsorbed species on the surface and the electrochemical potential. We demonstrate that, during the oxygen reduction reaction, hydroxyl intermediates on the cathode surface occur in several configurations with significantly different structures and reactivities. In particular, we find that near the open-circuit potential, non-hydrated hydroxyl is the dominant surface species. On the basis of density functional theory calculations, we show that the removal of hydration enhances the reactivity of oxygen species. Tuning the hydration of hydroxyl near the triple phase boundary will be crucial for designing more active fuel cell cathodes. The performance of polymer electrolyte membrane (PEM) fuel cells is limited by the sluggish kinetics of the oxygen reduction reaction (ORR) at the platinum (Pt) cathode. An improved understanding of catalytic steps of the ORR is thus essential for overcoming these limitations. Through electrochemical measurements, the ORR has been inferred to occur through a hydroxyl (OH) intermediate [1] , [2] . Indeed, based on density functional theory (DFT) simulations of the oxygenated intermediates of the ORR, it has been proposed that the Pt–OH bond strength could be a key descriptor of ORR activity and could therefore guide catalyst design [3] , [4] , [5] . However, recent experiments have observed unusual ORR activity in the presence of various ions [6] , [7] , in dehydrated environments [8] and on stepped surfaces with limited terrace widths [9] , [10] . These indicate that experiments to observe and characterize OH species directly during the ORR are essential. As most in situ experimental methods cannot detect oxygenated adsorbed species, the identification of OH is especially challenging. For example, Pt L -edge X-ray absorption spectroscopy, which probes the Pt substrate [11] , is typically sensitive to changes in the Pt oxidation state but cannot distinguish OH from other oxygenated species adsorbed on the surface [12] . The application of vibrational spectroscopy is also limited by the strong absorbance of both the electrolyte solution and the electrolyte membrane, which makes the weak vibrational signature of the OH species virtually undetectable [13] , [14] . X-ray photoelectron spectroscopy (XPS), which probes all oxygenated surface species with equal sensitivity, has been used to study Pt single-crystal electrodes [15] , [16] in ultra-high vacuum. The challenge with these ex situ measurements is to minimize decomposition and contamination during sample transfer, as surface water species on Pt all desorb above 200 K in ultra-high vacuum [17] . Here we report in situ identification of oxygenated intermediates on a Pt cathode during the ORR using ambient pressure XPS (APXPS), which enables measurements under high gas pressures (<100 Torr) [18] , [19] . We are able to identify the oxygenated intermediates of the ORR through their specific O 1 s chemical shifts. Using XPS studies of well-defined model systems as spectroscopic references, we differentiate two types of OH intermediates whose population depends on cell voltage: hydrated and non-hydrated OH. We also establish that non-hydrated OH is the dominant surface species on a Pt cathode during the ORR at high partial pressures of O 2(g) . With the assistance of DFT calculations, we show that the reduction of non-hydrated OH requires less overpotential than that of hydrated OH. This indicates that tuning OH hydration through cathode or electrolyte design will be crucial for enhancing ORR activity. Photoelectron spectroscopy measurements We designed a PEM fuel cell compatible with our APXPS system ( Fig. 1 ). To date, APXPS has been applied to the study of high-temperature solid-oxide fuel cells [20] but not to PEM fuel cells. In Fig. 2a , we show the O 1 s spectra and potentials of the cathode before and after the introduction of 0.4 Torr of O 2(g) under open-circuit conditions. The evolution of cell voltage as a function of time is further explained in Methods: Evolution of cell voltage and Supplementary Fig. S1 . Anodic charging following the introduction of O 2(g) causes the electrochemical potential at the cathode to increase from 0.1 to 0.9 V. The latter voltage of 0.9 V represents the maximum electrochemical potential available at the cathode in our set-up; the deviation from the Nernst potential of the ORR at the 0.4-Torr O 2 pressure (1.182 V) is attributed to kinetic losses [3] . For a given potential, the spectra recorded at different positions on the sample do not differ strongly, which indicates that the electrochemistry is not localized but occurs throughout the surface. This suggests that only a few layers of interfacial water are needed to conduct protons across the interface; recent studies of photocatalytic water splitting reached a similar conclusion [21] . 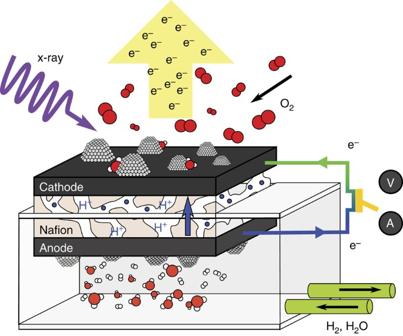Figure 1: Electrochemical cell for photoelectron spectroscopy. Schematic drawing of a PEM fuel cell set-up for APXPS investigations: the electrochemical cell has a Nafion membrane coated on both sides with a mixture of Nafion and carbon-supported Pt nanoparticles with catalyst loading of 4 mg cm−2(particle size 10–20 nm), which serve as anode and cathode. The cathode side of the assembly was exposed to the APXPS gas cell, which was filled with oxygen gas. The anode chamber was filled with humidified forming gas (95% N2/5% H2,saturated H2O). The voltmeter and galvanometer used for measurements are denoted by V and A, respectively. By connecting both electrodes to an external voltmeter or galvanometer, we can simultaneously record both XPS and either cell voltage or cell current. Figure 1: Electrochemical cell for photoelectron spectroscopy. Schematic drawing of a PEM fuel cell set-up for APXPS investigations: the electrochemical cell has a Nafion membrane coated on both sides with a mixture of Nafion and carbon-supported Pt nanoparticles with catalyst loading of 4 mg cm −2 (particle size 10–20 nm), which serve as anode and cathode. The cathode side of the assembly was exposed to the APXPS gas cell, which was filled with oxygen gas. The anode chamber was filled with humidified forming gas (95% N 2 /5% H 2, saturated H 2 O). The voltmeter and galvanometer used for measurements are denoted by V and A, respectively. By connecting both electrodes to an external voltmeter or galvanometer, we can simultaneously record both XPS and either cell voltage or cell current. 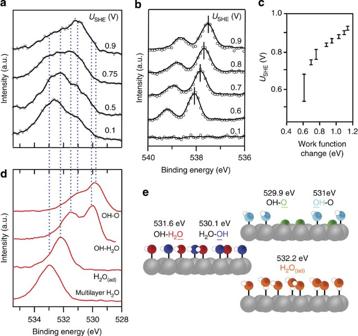Figure 2: Identification of oxygenated species on Pt cathode. (a) O 1sXPS spectra of a fuel cell cathode. The incident photon energy was 670 eV. Dots and solid lines correspond to experimental results and smoothened curves (first-order binomial), respectively. Spectra between 0.5 and 0.9 V were collected while exposing the anode to 600 Torr of humidified forming gas and the cathode to 0.4 Torr O2. The spectrum at 0.1 V was taken in the absence of oxygen. (b) O 1sXPS spectra of oxygen gas in the vicinity of the cathode. The electrochemical potential of the cathode quoted against standard hydrogen electrode (SHE),USHE, was measured simultaneously against the anode. The observed multiplet splitting is due to the coupling between the unpaired spins in the valence and core levels in a paramagnetic oxygen molecule33. (c) Plot of the measured cathode potential versus the change in work function. The bottom and top of bar correspond to the cathode electrochemical potential measured at the beginning and end of XPS data accumulation, respectively. (d) O 1sXPS spectra of oxygenated surface species on Pt(111). Bottom to top: multilayer H2O24; H2O(ad)24; adsorbed H2O-OH25; adsorbed OH-O measured in 0.05 Torr O2and 0.05 Torr H2at 450 K. (e) Schematic models and BE for oxygenated species: H2O(ad)(orange, 532.2 eV), H2O-OH (red, 531.6 eV), H2O-OH (blue, 530.1 eV), O-OH (cyan, 531 eV) andO-OH (green, 529.9 eV). Full size image Figure 2: Identification of oxygenated species on Pt cathode. ( a ) O 1 s XPS spectra of a fuel cell cathode. The incident photon energy was 670 eV. Dots and solid lines correspond to experimental results and smoothened curves (first-order binomial), respectively. Spectra between 0.5 and 0.9 V were collected while exposing the anode to 600 Torr of humidified forming gas and the cathode to 0.4 Torr O 2 . The spectrum at 0.1 V was taken in the absence of oxygen. ( b ) O 1 s XPS spectra of oxygen gas in the vicinity of the cathode. The electrochemical potential of the cathode quoted against standard hydrogen electrode (SHE), U SHE , was measured simultaneously against the anode. The observed multiplet splitting is due to the coupling between the unpaired spins in the valence and core levels in a paramagnetic oxygen molecule [33] . ( c ) Plot of the measured cathode potential versus the change in work function. The bottom and top of bar correspond to the cathode electrochemical potential measured at the beginning and end of XPS data accumulation, respectively. ( d ) O 1 s XPS spectra of oxygenated surface species on Pt(111). Bottom to top: multilayer H 2 O [24] ; H 2 O (ad) [24] ; adsorbed H 2 O-OH [25] ; adsorbed OH-O measured in 0.05 Torr O 2 and 0.05 Torr H 2 at 450 K. ( e ) Schematic models and BE for oxygenated species: H 2 O (ad) (orange, 532.2 eV), H 2 O -OH (red, 531.6 eV), H 2 O- O H (blue, 530.1 eV), O- O H (cyan, 531 eV) and O -OH (green, 529.9 eV). Full size image First, we establish the relationship between the electrochemical potential and surface species at the cathode. Both the electrochemical potential and the work function of a surface describe how strongly it binds electrons. It has been demonstrated that shifts in the XPS-binding energies (BE) of gaseous molecules, when referenced to the Fermi level in the vicinity of the surface [20] , [22] , can be used to determine changes in the work function; accordingly, changes in the electrochemical potential can be inferred from XPS. Guided by that principle, we measured the O 1 s XPS spectra of oxygen molecules in the vicinity of the cathode ( Fig. 2b ). From the shifts in the gas-phase peak, we were able to correlate changes in the work function with those in the cathode electrochemical potential ( Fig. 2c ). As these two sets of shifts closely agree, the observed changes in electrochemical potential at the cathode must arise from changes in surface speciation. To understand the relationship between electrochemical potential and surface species at the cathode, we compared our results with previously assigned XPS features of various oxygenated adsorbates on Pt. We compare our results to Pt(111), as our system contains nanoparticles 10–20 nm in size (see Methods) the close-packed terrace sites will dominate [23] . In Fig. 2d,e , we display O 1 s spectra and corresponding schematic illustrations for four oxygenated adsorbate systems on Pt(111): multilayer H 2 O [24] ; adsorbed H 2 O (H 2 O (ad) ) [24] ; co-adsorbed H 2 O and OH (H 2 O-OH) [25] ; co-adsorbed OH and O (OH–O). These reference spectra indicate that features at 533 and 532.2 eV are assigned to multilayer H 2 O and H 2 O (ad) , respectively. The co-adsorbed H 2 O-OH layer, in which both OH and H 2 O are hydrogen bonded to each other, yields O 1 s features at 531.6 and 530.1 eV arising from adsorbed water (H 2 O -OH) and OH (H 2 O- O H), respectively. The co-adsorbed OH–O layer, in contrast, gives rise to an OH feature at 531 eV ( O H-O) and a second feature at 529.9 eV that is assigned to adsorbed O on Pt(111) [25] (OH- O ); that the BE of OH is 0.9 eV higher in O H-O (non-hydrated OH) than in H 2 O- O H (hydrated OH) is attributed to the absence of hydrogen bonding in the former phase. Turning to Fig. 2d , with spectra measured in situ under open-circuit conditions, we see that water-related spectral features dominate at lower potentials (0.1 and 0.5 V). Under these conditions, we clearly resolve a low-binding energy shoulder arising from a hydrogen-bonded network of co-adsorbed OH and H 2 O species (H 2 O-OH). At high potentials (0.75 and 0.9 V), the dominant feature at 531 eV cannot be explained solely by hydrated OH, even when considering the 0.3 eV BE variation due to different facets [16] . Thus, we assign it to non-hydrated OH with small contribution from OH- O . The broadness of the spectra recorded at high potentials arises from the existence of OH species with differing degrees of hydration—the BE of OH ranges from 531 eV for non-hydrated OH to 530.1 eV for fully hydrated OH—as well as from the heterogeneity of the Pt nanoparticles in the sample. We now shift our focus to the role of adsorbates on the cathode when a current is extracted. 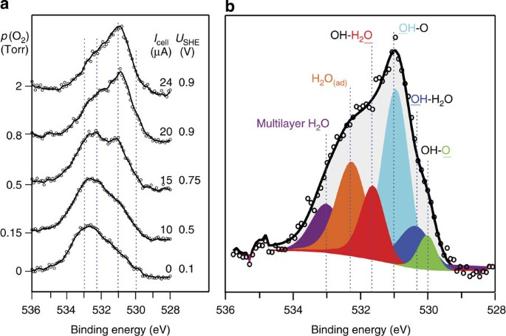Figure 3: XPS spectra of cathode under operating conditions. (a) O 1sXPS spectra obtained for an operating (closed circuit) fuel cell cathode. The incident photon energy was 670 eV. Spectra were collected under 600 Torr of humidified forming gas at the anode and varying O2pressures at the cathode, as shown. The resulting current outputs,Icell, and the elucidated cathode potential,USHE, measured using XPS (see Methods: Comparison of XPS spectra andSupplementary Fig. S2) are indicated. Dots correspond to experimental results and solid lines correspond to smoothened curves (first-order binomial). The spectral changes were reversible with respect top(O2). The blue dotted lines correspond to the model structures on Pt(111) discussed inFig. 2b. (b) Peak-fitted O 1sXPS spectrum in 0.8 Torr oxygen. The spectra were deconvoluted using Gaussian-broadened Doniach–Šunjić functions. Because of the large number of species and parameters, this peak fitting is more qualitative than quantitative in its nature, guiding the reader’s eye to the different surface species: multilayer H2O (purple), H2O(ad)(orange), H2O-OH (red),OH-O (cyan), H2O-OH (blue) and OH-O(green). Figure 3a shows the O 1 s spectra of the cathode surface collected while the cell is generating current (‘closed circuit’ conditions). These spectra were stable under constant O 2 pressure ( p (O 2 ), and their profiles were reversible with respect to variations of ( p (O 2 ). At low oxygen pressures ( p (O 2 )<0.15 Torr), multilayer H 2 O and H 2 O (ad) features dominate; the spectra recorded at oxygen pressures of 0 and 0.15 Torr are similar to the 0.1 and 0.5 V spectra shown in Fig. 2a obtained under open-circuit conditions (the elucidation of the cathode potential is described in Methods: Comparison of XPS spectra and Supplementary Fig. S2 ). As the O 2 pressure increases ( p (O 2 )>0.5 Torr), the current output increases and the spectra develop a major feature at a BE corresponding to non-hydrated OH species. Figure 3b illustrates this point by showing a spectral deconvolution of the surface species at an oxygen pressure of 0.8 Torr. Although this spectral decomposition is not unique because of the numerous species involved and the multiple degrees of hydrogen bonding available to the OH species, all fits agree that the most prominent spectral feature arises from non-hydrated OH. These results clearly identify that non-hydrated OH species is a key surface species of ORR. Figure 3: XPS spectra of cathode under operating conditions. ( a ) O 1 s XPS spectra obtained for an operating (closed circuit) fuel cell cathode. The incident photon energy was 670 eV. Spectra were collected under 600 Torr of humidified forming gas at the anode and varying O 2 pressures at the cathode, as shown. The resulting current outputs, I cell , and the elucidated cathode potential, U SHE , measured using XPS (see Methods: Comparison of XPS spectra and Supplementary Fig. S2 ) are indicated. Dots correspond to experimental results and solid lines correspond to smoothened curves (first-order binomial). The spectral changes were reversible with respect to p (O 2 ). The blue dotted lines correspond to the model structures on Pt(111) discussed in Fig. 2b . ( b ) Peak-fitted O 1 s XPS spectrum in 0.8 Torr oxygen. The spectra were deconvoluted using Gaussian-broadened Doniach–Šunjić functions. Because of the large number of species and parameters, this peak fitting is more qualitative than quantitative in its nature, guiding the reader’s eye to the different surface species: multilayer H 2 O (purple), H 2 O (ad) (orange), H 2 O -OH (red), O H-O (cyan), H 2 O- O H (blue) and OH- O (green). Full size image Theoretical simulations Using DFT and Monte Carlo simulations, we have calculated the coverages of adsorbed water (H 2 O (ad) ), OH (OH (ad) ) and O (O (ad) ) as a function of computed electrochemical potential ( Fig. 4a ). We emphasize that the coverages are averaged quantities. At low potentials, below 0.65 V, H 2 O (ad) is the dominant species. Above 0.65 V, OH (ad) begins to appear from the oxidation of H 2 O (ad) . Passing the reversible potential of this reaction at 0.76 V (ref. 26 ), the coverage of OH ( θ (OH (ad) ) becomes greater than that of H 2 O (ad) ( θ (H 2 O (ad) ). Higher potentials lead to further oxidation of OH (ad) into O (ad) , which becomes the dominant surface species at potentials above the reversible potential of 0.95 V (ref. 26 ). Representative snapshots of the adsorbate layer at two different potentials (0.8 and 0.95 V) are shown in Fig. 4b . First, we find that at 0.8 V, all OH (ad) have hydrogen bonds to H 2 O (ad) indicating only hydrated OH is present on the surface. On the other hand, we find OH (ad) both with and without hydrogen bonds to H 2 O (ad) at 0.95 V. This is consistent with the XPS results ( Fig. 2a ), which show that adsorbed water and hydrated OH prevail at low potentials, whereas non-hydrated OH appears at high potentials. The emergence of OH (ad) without hydrogen bond is correlated with the appearance of O (ad) -rich domains, which displace H 2 O (ad) because of repulsive interactions between O (ad) and H 2 O (ad) . Through this insight, we explain that the hydrated and non-hydrated OH observed in Fig. 3b co-exist in localized domains. 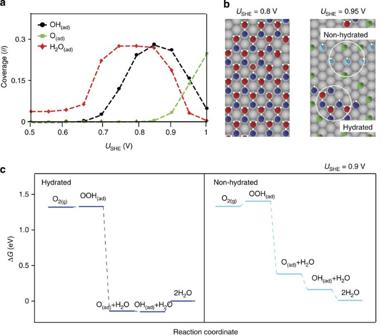Figure 4: DFT and Monte Carlo simulations. (a) Calculated coverages of adsorbed oxygen, OH and water as a function of computed electrochemical potential,USHE, obtained from DFT and Monte Carlo simulations. The regions marked are separated by the emergence of O(ad)at 0.85 V. (b) Representative snapshots of the surface at 0.8 and 0.95 V from the Monte Carlo simulations exemplify the two regimes shown ina, with H2O(ad)(red and white circles), hydrated OH(ad)(blue and white circles), non-hydrated OH(ad)(cyan and white circles) and O(ad)(green circles) shown on a Pt (grey circles) surface. The adsorbate layer between 0.85 and 1 V consists of co-existing localized domains of both hydrated and non-hydrated OH, which we have marked in the corresponding schematic. (c) Free-energy diagrams for the ORR, based on DFT calculations for both hydrated and non-hydrated pathways, at a potential ofUSHE=0.9 V. The change in Gibbs free energy, ΔG, along the reaction coordinate shows that the thermodynamically limiting step in the hydrated phase is the removal of adsorbed OH. In the non-hydrated phase, the limiting step is the activation of O2as OOH(ad). Figure 4: DFT and Monte Carlo simulations. ( a ) Calculated coverages of adsorbed oxygen, OH and water as a function of computed electrochemical potential, U SHE , obtained from DFT and Monte Carlo simulations. The regions marked are separated by the emergence of O (ad) at 0.85 V. ( b ) Representative snapshots of the surface at 0.8 and 0.95 V from the Monte Carlo simulations exemplify the two regimes shown in a , with H 2 O (ad) (red and white circles), hydrated OH (ad) (blue and white circles), non-hydrated OH (ad) (cyan and white circles) and O (ad) (green circles) shown on a Pt (grey circles) surface. The adsorbate layer between 0.85 and 1 V consists of co-existing localized domains of both hydrated and non-hydrated OH, which we have marked in the corresponding schematic. ( c ) Free-energy diagrams for the ORR, based on DFT calculations for both hydrated and non-hydrated pathways, at a potential of U SHE =0.9 V. The change in Gibbs free energy, Δ G , along the reaction coordinate shows that the thermodynamically limiting step in the hydrated phase is the removal of adsorbed OH. In the non-hydrated phase, the limiting step is the activation of O 2 as OOH (ad) . Full size image Our studies not only confirm the presence of OH (ad) during ORR conditions but, most importantly, also demonstrate that there are two phases of OH, hydrated OH and non-hydrated OH, co-existing under operating conditions. This distinction led us to evaluate their reactivity for the reduction of oxygen by constructing a free-energy diagram at a potential of 0.9 V based on DFT calculations ( Fig. 4c ). In the hydrated pathway, the limiting step is associated with the removal of OH (ad) on Pt(111). In the non-hydrated pathway, the removal of hydration enhances the reactivity of OH (ad) but creates a thermodynamic barrier to the activation of O 2(g) as adsorbed OOH (OOH (ad) ) because of a combination of weakening interactions from dehydration and repulsive adsorbate–adsorbate interactions with O (ad) . Therefore, at 0.9 V, the thermodynamic barrier associated with the overall ORR process is 0.07 eV in the non-hydrated pathway, corresponding to the conversion of O 2(g) to OOH (ad) . On the other hand, in the hydrated pathway, this barrier becomes 0.15 eV for the removal of hydrated OH (ad) . This analysis suggests that extending the stability range of the non-hydrated phase will prove beneficial in improving the overall ORR activity. The importance of non-hydrated OH for the ORR at high potentials explains the enhanced ORR activity of Pt in hydrophobic ionic liquids [8] , in the presence of certain aqueous ions [6] , [7] and on stepped surfaces with narrow terrace width [9] , [10] . The last is unexpected as step sites strongly bind OH, as indeed observed with a reduced activity for small Pt nanoparticles [27] . However, whereas adsorbed H 2 O and OH form an extended hydrogen-bonding network on wide terraces [25] , that process is hindered on narrow terraces because of limited space and thus the amount of non-hydrated OH is increased. In general, dehydrated environments [8] will by their very nature limit the hydration of any OH intermediates. Finally, as hydrogen bonding of H 2 O to OH can compete with direct ion–OH interactions [28] , specific ions in the electrolyte could limit the hydration of OH [6] , [7] . This new insight into the subtle interplay between non-covalent hydrophobic and hydrophilic interactions can inspire the design of new catalysts, not only for the ORR but also for other relevant electrochemical reactions. Experimental details The electrochemical cell assembled on a polyetheretherketone (PEEK) polymer framework has a Nafion 115 membrane coated on both sides with Pt nanoparticles, which serve as anode and cathode, supported on a Nafion/carbon-black mixture with catalyst loading of 4 mg cm −2 from the Fuel Cell Store, Inc (Boulder, CO; particle size 10–20 nm). The cathode was exposed to the APXPS gas cell, which was filled with oxygen gas. The anode chamber was filled with humidified forming gas (95% N 2 /5% H 2 ) to provide hydrogen fuel and membrane humidification. For open-circuit measurements, the anode was used as a hydrogen electrode. All reported potentials are referenced to the standard hydrogen electrode. Using the Nernst equation, , the anode potential is calculated to be 0.065 V against standard hydrogen electrode. Here F is the Faraday constant, R is the universal gas constant, T is the temperature, p (H 2 ) is the partial pressure of hydrogen in the anode chamber and p 0 is the standard pressure. The XPS measurements were performed by placing the electrochemical cell into the gas cell of the APXPS system on beamline 13-2 at the Stanford Synchrotron Radiation Lightsource [19] . Water vapour and hydrogen were introduced through small tubes while the cathode side exposed in the gas cell was pressurized via variable leak valves. The XPS BE is referenced to the Fermi level through measurements of the valence band under the corresponding experimental conditions. Supplementary Figure S3 shows an overview XPS spectrum of the cathode surface together with inserts showing the detailed F 1 s and C 1 s spectra before and after the introduction of oxygen to the cathode. In addition to Pt and adsorbed oxygenated species, there are spectral features from water and fluorinated carbon in Nafion binder and carbon black. The sulphur spectral contributions from the Nafion region are small compared with the carbon-black region ruling out the involvement of sulphur-containing oxygenated species in the spectral changes. To rule out the contributions of either polymer or oxidized carbon black in the O 1 s spectra, we show the C 1 s and F 1 s XPS before and after the introduction of oxygen as the inset of Supplementary Fig. S3 , which indicate no increase of oxidized carbon- or fluorine-containing species. Evolution of cell voltage Supplementary Figure S1 shows the evolution of the cathode potential as a function of time under the open-circuit potential conditions in which the O 1 s XPS spectra shown in Fig. 2a were collected. The anode was supplied with 600 Torr of humidified forming gas, which also humidified the cathode through the diffusion of water across the Nafion membrane. At time t =0 min, we introduced 0.4 Torr of oxygen gas to the cathode chamber. After the introduction of the oxygen, the cathode potential increased, eventually maintaining a constant value of ~0.9 V. The development of cell voltage correlates well with the O 1 s changes in XPS of the cathode, as illustrated in the accompanying spectra ( t =5, 12, 130 and 177 min are also shown in Fig. 2a ). We note that no spectral change was observed after the cell potential reaches the constant value of 0.9 V. Comparison of XPS spectra Supplementary Figure S2 compares the O 1 s XPS spectra shown in Fig. 3a measured under closed-circuit conditions and the O 1 s XPS spectra shown in Fig. 2a measured under open-circuit conditions. The cathode operating at O 2 pressure of 0.15 Torr exhibits the same surface species as a cathode at an open-circuit potential of 0.1–0.5 V. On the other end, on the cathode at O 2 pressure above 0.8 Torr exhibits the same surface species as those observed at an open-circuit potential of 0.9 V. We used this information to elucidate the cathode potential under closed-circuit reaction conditions. Computational details The simulation of the reaction kinetics is accomplished through a combination of equilibrium and dynamic Monte Carlo methods using kinetic and thermodynamic parameters calculated from DFT. The DFT calculations were performed using the DACAPO and ASE codes ( https://www.wiki.fysik.dtu.dk ). The ionic cores were described using ultrasoft pseudopotentials [29] and the Kohn–Sham one-electron states were expanded using plane waves with kinetic energies below 340 eV. The density was expanded using plane waves with a cutoff corresponding to 500 eV and the first Brillouin zone was sampled using a 4 × 4 × 1 mesh of Monkhorst–Pack k -points [30] . The Hamiltonian was corrected for the electrostatic dipole interaction between periodically repeated slabs [31] . A lattice-gas model was employed in the Monte Carlo simulations, which treats the hydrogen bonding between different water species, OH and O. The interaction energies between various species are summarized in Supplementary Table S1 . A full description of the methodology is given in ref. 26 . The free-energy diagram for the reduction of O 2 to H 2 O in the hydrated environment is based on DFT calculations from ref. 32 . The free-energy diagram for O 2 reduction in the O-rich non-hydrated environment is calculated based on DFT calculations by combining corrections to the adsorbate due to the H 2 O and O environment separately as described below. The free-energy non-hydrated OH is derived from a 0.26 eV destabilization of OH based on differences in OH–H 2 O interactions in hydrated and non-hydrated environments [26] . In addition, a 0.04 eV destabilization of OH adsorbed on top is found for OH co-adsorbed with 1/4 monolayer (ML) of O. The free energy of O in the non-hydrated environment is calculated from a 0.51-eV destabilization of O with 1/4 ML of O co-adsorbed. The interaction between O and H 2 O is weak [3] and differences in H 2 O–O interactions have been neglected for the free energy of O. The free energy of OOH is obtained from a 0.05 eV destabilization from 1/4 ML of O and a 0.02 eV destabilization of OOH in a pure H 2 O environment compared with an OH/H 2 O environment. The calculation of the interactions between O and OOH, O and O, OH and O and the water stabilization of OOH are all performed in a surface unit cell. All computational cells contained four Pt(111) layers where the bottom two layers are fixed in their bulk positions. The geometry of the two topmost Pt layers and adsorbates is optimized until the largest force component is below 0.03 eV Å −1 . The electrochemical potentials were calculated using the computational hydrogen electrode method [3] . How to cite this article: Casalongue, H. S. et al . Direct observation of the oxygenated species during oxygen reduction on a platinum fuel cell cathode. Nat. Commun. 4:2817 doi: 10.1038/ncomms3817 (2013).